Analysis of clinically relevant variants from ancestrally diverse Asian genomes Asian populations are under-represented in human genomics research. Here, we characterize clinically significant genetic variation in 9051 genomes representing East Asian, South Asian, and severely under-represented Austronesian-speaking Southeast Asian ancestries. We observe disparate genetic risk burden attributable to ancestry-specific recurrent variants and identify individuals with variants specific to ancestries discordant to their self-reported ethnicity, mostly due to cryptic admixture. About 27% of severe recessive disorder genes with appreciable carrier frequencies in Asians are missed by carrier screening panels, and we estimate 0.5% Asian couples at-risk of having an affected child. Prevalence of medically-actionable variant carriers is 3.4% and a further 1.6% harbour variants with potential for pathogenic classification upon additional clinical/experimental evidence. We profile 23 pharmacogenes with high-confidence gene-drug associations and find 22.4% of Asians at-risk of Centers for Disease Control and Prevention Tier 1 genetic conditions concurrently harbour pharmacogenetic variants with actionable phenotypes, highlighting the benefits of pre-emptive pharmacogenomics. Our findings illuminate the diversity in genetic disease epidemiology and opportunities for precision medicine for a large, diverse Asian population. Genomics is increasingly an integral part of mainstream medicine and has the potential to revolutionize healthcare delivery globally [1] . A critical enabler of precision medicine is the availability of genomic variation data from both patients and the general population, to accurately assess whether a variant is disease-causing and to identify genetic disorders prevalent in the population [2] . Despite advances in genomics research, persistent Eurocentric biases in sequencing studies have resulted in inequitable access to precision medicine [3] , [4] , [5] . Although comprising nearly 60% of the global population, Asian genomes are relatively scarce; for example, constituting 6.6% of the widely-used Genome Aggregation Database (gnomAD, v3.1) and 3% of population health studies [6] , [7] . Despite the diversity among Asians [8] , nearly all Asian genomes in population databases are of East and South Asian ancestry, with severe under-representation of Southeast Asians. Increasing Asian representation in the characterization of medically relevant population genetic data is crucial to address several disparities that affect a large global population. First, healthcare professionals serving non-European populations may be less aware of genetic disorders and associated symptoms in their patients, increasing risk of misdiagnosis or mistreatment [9] . Second, carrier screening panels are mostly derived from European-descent populations and may miss genetic disorders common in non-Europeans. Finally, bias in submissions to variant databases leads to the clinical interpretation of rare variants in non-Europeans being more challenging, reducing the likelihood of reporting and perpetuating the lack of publicly available information [10] , [11] . Emerging work on diverse populations is also highlighting complex relationships between self-reported and genetically-inferred ancestry, reflecting the importance of considering admixture when evaluating personalized genetic risk [12] . This is relevant given the spread and integration of the Asian diaspora with other continental populations. Singapore, a Southeast Asian city-state of four million residents [13] , has a diverse population comprising three major ethnic groups: Chinese (74.2%), Malay (13.7%), Indian (8.9%) of East Asian, Southeast Asian, and South Asian ancestry, respectively. Population-scale sequencing of Singaporean genomes is thus a particularly attractive effort [14] to provide insights into genetic disease risk and to address knowledge gaps for populations across East Asia, South Asia, and a major proportion of Austronesian-speaking Southeast Asian group represented by Malays. Here, we perform deep interrogation of clinically significant genetic variants from 9051 Singaporean whole genomes and characterize (1) prevalence of autosomal dominant (AD) disorders, (2) carrier frequency of autosomal recessive (AR) and X-linked conditions, and (3) evaluate distribution of pharmacogenomic variation across the three ancestry groups. We also examine the implications of genetic admixture on personalized disease risk in this ancestry-diverse population. Our findings demonstrate the diversity of genetic epidemiology of disease in multi-ethnic Asian populations and highlight opportunities for coupling genetic disease risk profiling with pre-emptive pharmacogenomics for therapy optimization. 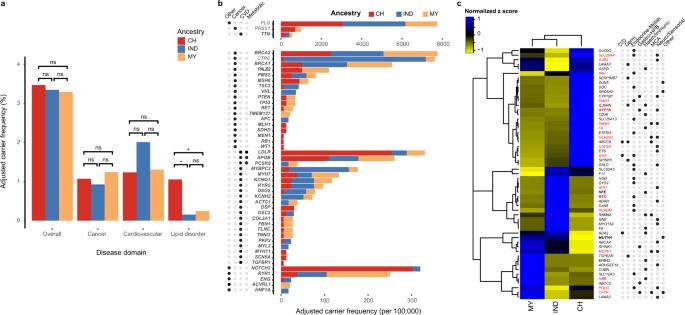Fig. 1: Spectrum of pathogenic variation in clinically relevant genes among Singaporeans. aCarrier frequencies of ACMG SF v3.0 genes associated with dominant disorders compared across the three main ancestry groups. The disorders are further sub-classified into three main disease domains for comparison (cancer, cardiovascular, lipid disorders). Carrier frequency of P/LP variants in lipid disorder genes were significantly higher among Chinese compared to Indians (p= 7.93 × 10−5) and Malays (p= 1.70 × 10−3). Statistical significance was evaluated by two-sided Fisher’s exact test, with Benjamini-Hochberg correction for multiple testing. Adjustedp< 0.05 was considered significant, ns: not significant. CH: Chinese, IND: Indian, MY: Malay.bDifferential distribution of carrier frequencies across ancestries for dominantly inherited genetic disorders associated with ACMG SF v3.0 medically actionable genes, or non-ACMG SF v3.0 genes with a carrier frequency >0.5%.cGenes of recessive conditions with significant differences in carrier frequency of P/LP variants across ancestry groups. Colour scale maps to row-wise z-scores, obtained by subtracting from each gene-level carrier frequency the row average and then dividing the value by the row standard deviation. Genes in red fonts are recommended by ACMG for carrier screening. Genes in bold fonts are part of the ACMG SF v3.0 list. The disorder domain associated with pathogenic alteration of the indicated gene is represented in the dot matrix. CVD cardiovascular disorders, Derm dermatological disorders, Metab. metabolic (including lysosomal storage, mitochondrial, metabolic disorders), Gastro-HPB gastro-hepato-pancreato biliary disorders, Haem/Immuno haematological/immunological disorders, MCA multiple congenital anomalies, Neuro neurological (including neurologic, neuromuscular, neurodegenerative disorders), Others: including cancer, respiratory, genitourinary disorders. Study characteristics Our analysed cohort of 9,051 individuals from SG10K_Health project is a cross-section of the Singaporean population, inferred to be unrelated to the second degree (Supplementary Table 1 ). 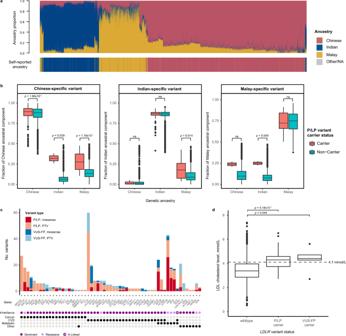Fig. 2: Evaluating the influence of genetic admixture and potentially pathogenic VUS in SG10K_Health cohort. aADMIXTURE analysis of inferred genetic ancestral components at K = 3 juxtaposed with self-reported ancestry for the 9,051 Singaporean individuals. NA: not available.bThe proportion of genetic ancestral components tracked consistently with carrier status of pathogenic/likely pathogenic (P/LP) variants specific to the associated ancestry group across Singaporean Chinese (CH), Indian (IND) and Malay (MY) individuals (Chinese-specific variant carriers/non-carriers: (CH) 455/5047, (IND) 2/1939, (MY) 26/1582; Indian-specific variant carriers/non-carriers: (CH) 3/5499, (IND) 147/1794, (MY) 19/1589; Malay-specific variant carriers/non-carriers: (CH) 2/5500, (IND) 2/1939, (MY) 24/1584). Pairwise differences between carriers and non-carriers were evaluated by two-sided Wilcoxon rank-sum test.p< 0.05 was considered significant. ns: not significant.cJuxtaposition of P/LP variants with potentially pathogenic variants of uncertain significance (missense and cryptic splice variants) classified as VUS-FP, identified in genes from the ACMG SF v3.0 list. Mode of inheritance and disease domain associated for each gene are indicated in the dot matrix below. PTV: protein-truncating variant.dCarriers of VUS-FP variants (n= 5) identified inLDLRdemonstrated LDL cholesterol range that is consistent with carriers of P/LP variants (n= 25) and is higher compared to non-carriers (n= 4397). An LDL cholesterol level of ≥4.1 mmol/L is classified as high by the Ministry of Health Singapore.pvalues were derived from binomial logistic regression comparing LDL cholesterol levels againstLDLRvariant status, correcting for age, sex, genetic ancestry, and lipid-lowering medication intake. All box plots extend from the 25th to 75th percentiles and the length of the whiskers are defined as follows: upper whisker =  min(maximum_value, Q3 + 1.5*IQR), lower whisker = max(mininum_value, Q1–1.5*IQR), where IQR is interquartile range, Q3 is third quartile, Q1 is first quartile. Horizontal line in the box represents the median. Individual age ranged between birth-85 years (median: 47 years) and comprised 57.3% females (Supplementary Table 2 ). Using ADMIXTURE (ver 1.3.0) [15] , we inferred genetic ancestry of individuals, who were mostly Chinese (60.8%) followed by Indian (21.4%) and Malay (17.8%). Whole genome sequences were jointly analysed and variants occurring in 4,143 genes associated with AD, AR and X-linked monogenic disorders were curated according to the American College of Medical Genetics and Genomics (ACMG) guidelines and classified according to a standardized workflow (Supplementary Fig. 1 ). Overall, we identified 4,960 pathogenic/likely pathogenic (P/LP) single nucleotide variants and micro-indels, of which 82.2% were protein-length changes, as well as 406 gross deletions in loss-of-function intolerant (LOFi) genes. Prevalence of variants associated with autosomal dominant disorders We identified 238 (2.63%) individuals harbouring at least one of the 163 P/LP variants identified in 35 dominant condition genes of the ACMG secondary findings (SF) v2.0 gene list (Supplementary Data 1 , 2 ), the prevalence of which is comparable to reported yields of 1.86% to 2.85% in smaller East Asian cohorts [16] , [17] and 2.0% to 2.54% predominantly European cohorts [18] , [19] . This yield increased to 3.41% with the expanded ACMG SF v3.0 list, identifying an additional 71 individuals, most of whom are protein-truncating variant carriers in the newly included cardiomyopathy gene TTN (53/71) and hereditary breast and ovarian cancer (HBOC) syndrome gene PALB2 (11/71). Only two individuals (2/309) had P/LP variants in multiple genes: one harbouring predisposition to familial hypercholesterolemia (FH) and long QT syndromes ( PCSK9, KCNH2 ) and the other with predisposition to cancer and hypertrophic cardiomyopathy ( SDHD , MYBPC3 ). Although the overall prevalence of AD disorder variants across ancestry groups was similar ( p > 0.05), concentration of genetic risk was unequal for certain disease domains (Fig. 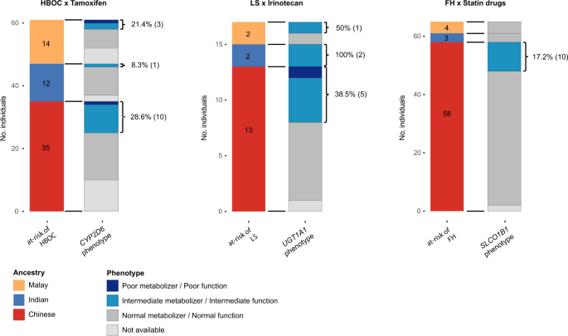Fig. 3: Carriers of both germline pathogenic/likely pathogenic (P/LP) variant in a CDC Tier 1 condition and pharmacogenetic variant associated with an actionable phenotype to drugs used for treatment. Only pharmacogenetic variant-drug combinations supported by PharmGKB Level 1A/1B evidence were considered. HBOC hereditary breast and ovarian cancer syndrome, LS Lynch syndrome, FH familial hypercholesterolemia,nnumber of germline P/LP variant carriers for the indicated CDC Tier 1 genetic conditions among 9051 Singaporeans. 1a , Supplementary Table 3 ). Notably, we observed significantly higher genetic risk for FH among Chinese (1.05%) compared to Indians (0.15%, p = 7.93 × 10 −5 ) and Malays (0.25%, p = 1.70 × 10 −3 ), predominantly driven by LDLR carriers among Chinese (0.76%, Table 1 ). While genetic risk for cancer and cardiovascular disorders were not significantly different across the three ancestry groups, we found ancestry-specific distinctions at the variant level. For instance, carrier frequency for P/LP variants in the hypertrophic cardiomyopathy gene MYBPC3 was eight-fold higher among Indians (0.41%) compared to Chinese (0.05%), attributed to the significantly higher frequency of MYBPC3 c.1790G > A (p.Arg597Gln) variant (Indian: 0.31% vs Chinese: 0%, p = 9.38 × 10 −4 ). We also observed significantly higher carrier frequency of a known Malay founder variant associated with HBOC [20] , BRCA1 c.2726dup (p.Asn909Lysfs*6) among Malays in our study (0.25%, p = 0.032) compared to Chinese (0.02%) (Supplementary Fig. 2 ). To account for potential survivorship bias in our observation, we quantified carrier frequencies for our cohort subset aged ≤ 50 years and found that these ancestry-specific distinctions remain significant (Supplementary Data 3 ). Fig. 1: Spectrum of pathogenic variation in clinically relevant genes among Singaporeans. a Carrier frequencies of ACMG SF v3.0 genes associated with dominant disorders compared across the three main ancestry groups. The disorders are further sub-classified into three main disease domains for comparison (cancer, cardiovascular, lipid disorders). Carrier frequency of P/LP variants in lipid disorder genes were significantly higher among Chinese compared to Indians ( p = 7.93 × 10 −5 ) and Malays ( p = 1.70 × 10 −3 ). Statistical significance was evaluated by two-sided Fisher’s exact test, with Benjamini-Hochberg correction for multiple testing. Adjusted p < 0.05 was considered significant, ns: not significant. CH: Chinese, IND: Indian, MY: Malay. b Differential distribution of carrier frequencies across ancestries for dominantly inherited genetic disorders associated with ACMG SF v3.0 medically actionable genes, or non-ACMG SF v3.0 genes with a carrier frequency >0.5%. c Genes of recessive conditions with significant differences in carrier frequency of P/LP variants across ancestry groups. Colour scale maps to row-wise z-scores, obtained by subtracting from each gene-level carrier frequency the row average and then dividing the value by the row standard deviation. Genes in red fonts are recommended by ACMG for carrier screening. Genes in bold fonts are part of the ACMG SF v3.0 list. The disorder domain associated with pathogenic alteration of the indicated gene is represented in the dot matrix. CVD cardiovascular disorders, Derm dermatological disorders, Metab. metabolic (including lysosomal storage, mitochondrial, metabolic disorders), Gastro-HPB gastro-hepato-pancreato biliary disorders, Haem/Immuno haematological/immunological disorders, MCA multiple congenital anomalies, Neuro neurological (including neurologic, neuromuscular, neurodegenerative disorders), Others: including cancer, respiratory, genitourinary disorders. Full size image Table 1 Consolidated top 10 autosomal dominant and autosomal/X-linked recessive disorder genes with highest carrier frequencies of P/LP variants identified in each ancestry group in Singapore Full size table Beyond ACMG SF v3.0 genes, we identified four AD genes ( FLG , NOTCH3 , PRSS1 , CTRC ) with carrier frequencies exceeding 0.5% in at least one ancestry group (Table 1 ). These genes are either associated with non-life-threatening disorders ( FLG ; ichthyosis vulgaris), late-onset disorders ( NOTCH3 ; cerebral autosomal dominant arteriopathy with sub-cortical infarcts and leukoencephalopathy, CADASIL) or risk factors for disease ( PRSS1 , CTRC ; hereditary pancreatitis). Genetic risk differed across ancestry groups for these genes (Fig. 1b ), primarily driven by ancestry-specific recurrent variants. For instance, CADASIL risk among Chinese stems from a recurrent NOTCH3 c.1630C > T (p.Arg544Cys) variant (0.91%) also prevalent among Taiwanese [21] , whereas the underlying genetic risk for hereditary pancreatitis differed between Chinese and Indians, contributed by a Chinese-predominant PRSS1 c.623G > C (p.Gly208Ala) variant (1.94%) and Indian-specific CTRC c.217G > A (p.Ala73Thr) variant (0.98%), respectively (Supplementary Data 2 ). Overall, carrier frequencies for genes with burden exceeding 0.5% in Chinese or Indians correlated well with frequencies in gnomAD East Asian and South Asian populations respectively (Supplementary Fig. 3 , Pearson’s r = 0.93, p = 3.8 × 10 −22 ). Next, we evaluated the population carrier burden of recessive conditions. Among AR genes, high carrier burden was observed for GJB2 , CFTR , and HFE (Table 1), each driven by elevated carrier frequencies in specific variants that confer milder disease. For instance, we detected a predominant GJB2 variant among Chinese and Malays; c.109G > A (p.Val37Ile; Chinese:18.5%, Malay:15.1%), known to be associated with mild-to-moderate hearing impairment [22] , whereas the HFE c.187C > G (p.His36Asp) variant identified recurrently among Indians (16.6%) has rarely been associated with frank clinical hemochromatosis although the variant is linked to biochemical abnormalities [23] . Despite high CFTR carrier burden, the variants with high carrier frequencies, c.4056G > C (p.Gln1352His) and c.1210-11T > G, are associated with congenital bilateral absence of vas deferens (CBAVD) and pancreatitis instead of cystic fibrosis. Nevertheless, we observed a few genes with high carrier burden that are driven by high carrier frequencies in known causal variants for disorders, such as the significant burden of SLC25A13 in Chinese (2.29%, p = 2.51 × 10 −14 ) due to a high carrier frequency of citrin deficiency-linked variant SLC25A13 c.852_855del (p.Met285Profs*2) [24] , [25] (Chinese: 1.45%) and GNE in Indians (3.40%, p < 9.6 x 10 -8 )  attributed to the GNE myopathy-linked c.2086G>A (p.Val696Met) variant [26] (Indian: 3.40%). Comparing disease risk profiles across ancestry groups, we observed distinctions attributable to highly recurrent variants in different genes (Fig. 1c ). Among Malays, who are unrepresented in existing population databases, we found higher carrier burden for beta-thalassemia, contributed by the common Southeast Asian HBB c.79G > A (p.Glu27Lys; 6.72% Malays), and retinopathies driven by recurrent variants in retinopathy-related genes ABCA4 (Stargardt disease, c.71G > A (p.Arg24His), 2.36%) and ARHGEF18 (retinitis pigmentosa, c.826-1G > A, 1.80%). Enriched among Chinese were recurrent variants in immune-related disorders, namely platelet glycoprotein IV deficiency-associated CD36 c.332_333del (p.Thr111Serfs*22, 3.29%) and generalized pustular psoriasis-linked IL36RN c.115 + 6 T > C (3.18%), as well as Krabbe leukodystrophy-associated GALC c.1901T > C (p.Leu634Ser, 1.15%); all of which are prevalent disease-associated variants reported in East Asian populations [27] , [28] , [29] . In Indians, we observed a high carrier frequency of factor V deficiency-associated F5 ‘Leiden’ c.1601G > A (p.Arg534Gln) variant (2.27% Indians) and a high carrier burden in BTD (7.42% Indians), which is predominantly driven by c.1270G > C (p.Asp424His; 6.80% Indians), a known mild variant that causes partial biotinidase deficiency in conjunction with another severe BTD variant [30] . Other recessive genes with carrier frequencies exceeding 1% include those associated with Pompe disease ( GAA ), Shwachman-Diamond syndrome ( SBDS ), EYS -associated retinitis pigmentosa, Gitelman syndrome ( SLC12A3 ), and DUOX2 -associated congenital hypothyroidism (Supplementary Data 1 ). Gaps in carrier screening panels for Asians Next, we evaluated the coverage of existing carrier screening panel recommendations against our population carrier burden of recessive conditions. We identified 70 recessive genes with carrier frequencies exceeding 0.5% in at least one ancestry (Supplementary Data 1 ), of which 21 genes are recommended by ACMG for carrier screening [31] , a further 18 genes are covered by commercial carrier screening panels, and the remaining 31 genes provided scope for expansion of carrier screening panels to better represent genetic disorders in Asian populations. Among the 70 genes, 37 are associated with severe recessive diseases, defined as “conditions with lethality in childhood, are significantly disabling or have a negative impact on quality of life for an affected child and the family” [32] . Ten of these 37 genes (27%) warranted inclusion but are not found in commercial carrier screening panels. These genes are associated with metabolic ( DDC, GYS2 ), cardiovascular ( ABCC6 ), developmental ( SBDS ), neurodegenerative ( ADAR ), ocular ( ABCA4 ), respiratory ( DNAH11 ), gastroenterologic ( CYP7B1 ), immunological ( ADA2 ) and dermatological ( SPINK5 ) disorders. Additionally, we estimated the proportion of couples in each ancestry group potentially at risk of having offspring affected by AR disorders (at-risk couples, ARCs) by exhaustively simulating all possible matings and then identifying instances where both partners in a theoretical pairing carry a P/LP variant in the same gene. Considering only 1,300 genes that cause severe recessive disorders [32] , we detected ARC proportions of 0.70%, 0.56%, and 0.51% in Malays, Indians and Chinese, respectively. Gross deletions in loss-of-function intolerant (LOFi) genes To determine the contribution of gross deletions to genetic disease risk, we identified pathogenic deletions between 500 bases to 10 megabases (Mb) affecting biologically relevant transcripts of LOFi genes. We found clinically significant deletions affecting SMN1 (AR spinal muscular atrophy) in 1.92% (37/1,923) of individuals and the 19 kb HBA1/HBA2 SEA deletion linked to alpha-thalassemia at a carrier frequency of 1.16% (Supplementary Data 4 ). We also detected a 2.9 kb deletion in AGT (AR renal tubular agenesis) previously reported as a Taiwanese founder mutation [33] and a 3.2 kb deletion in CLMP (AR congenital short bowel syndrome) in 0.61% and 0.20% of Chinese individuals, respectively. Among Indians, recurrent pathogenic deletions include CNGA1 (15 kb deletion, retinitis pigmentosa, 0.31%) and ALMS1 (1.3 kb deletion, Alström syndrome, 0.16%), whereas pathogenic deletions found in Malays include IFT140 (4.2 kb deletion, Mainzer-Saldino syndrome, 0.31%) and SLURP1 (32 kb deletion, Mal de Meleda, 0.31%). Genetic ancestry mapping reveals limitations of self-reported race/ethnicity (R/E) The use of self-reported R/E for evaluating genetic disease risk has implications in a multi-ethnic population such as Singapore because it is a social construct that does not reliably capture one’s genetic ancestry. To assess this effect, we compared population demography defined by self-reported R/E (captured in individual national identification document) with genetic ancestry inferred using ADMIXTURE fitted to three hypothetical ancestral components (K = 3), which recapitulated the three major ancestry groups in SG10K_Health (Fig. 2a ). Two groups emerged; individuals whose self-reported R/E was inconsistent (‘R/E-mismatched group’, n = 268, Supplementary Table 4 ) or consistent (‘R/E-matched group’, n = 8783) with the predominant ancestral component assigned by ADMIXTURE. Using the highest ancestral component proportion, maxQ, as a measure of admixture (with lower maxQ indicating higher admixture), we found that the R/E-mismatched group had significantly lower median maxQ compared to R/E-matched group (0.53 vs. 0.87, p = 1.93 × 10 −89 ), implying that recent admixture (e.g., mixed parentage), may be prevalent among R/E-mismatched individuals (Supplementary Fig. 4 ). Fig. 2: Evaluating the influence of genetic admixture and potentially pathogenic VUS in SG10K_Health cohort. a ADMIXTURE analysis of inferred genetic ancestral components at K = 3 juxtaposed with self-reported ancestry for the 9,051 Singaporean individuals. NA: not available. b The proportion of genetic ancestral components tracked consistently with carrier status of pathogenic/likely pathogenic (P/LP) variants specific to the associated ancestry group across Singaporean Chinese (CH), Indian (IND) and Malay (MY) individuals (Chinese-specific variant carriers/non-carriers: (CH) 455/5047, (IND) 2/1939, (MY) 26/1582; Indian-specific variant carriers/non-carriers: (CH) 3/5499, (IND) 147/1794, (MY) 19/1589; Malay-specific variant carriers/non-carriers: (CH) 2/5500, (IND) 2/1939, (MY) 24/1584). Pairwise differences between carriers and non-carriers were evaluated by two-sided Wilcoxon rank-sum test. p < 0.05 was considered significant. ns: not significant. c Juxtaposition of P/LP variants with potentially pathogenic variants of uncertain significance (missense and cryptic splice variants) classified as VUS-FP, identified in genes from the ACMG SF v3.0 list. Mode of inheritance and disease domain associated for each gene are indicated in the dot matrix below. PTV: protein-truncating variant. d Carriers of VUS-FP variants ( n = 5) identified in LDLR demonstrated LDL cholesterol range that is consistent with carriers of P/LP variants ( n = 25) and is higher compared to non-carriers ( n = 4397). An LDL cholesterol level of ≥4.1 mmol/L is classified as high by the Ministry of Health Singapore. p values were derived from binomial logistic regression comparing LDL cholesterol levels against LDLR variant status, correcting for age, sex, genetic ancestry, and lipid-lowering medication intake. All box plots extend from the 25th to 75th percentiles and the length of the whiskers are defined as follows: upper whisker =  min(maximum_value, Q3 + 1.5*IQR), lower whisker = max(mininum_value, Q1–1.5*IQR), where IQR is interquartile range, Q3 is third quartile, Q1 is first quartile. Horizontal line in the box represents the median. Full size image Given admixture in the population, it is conceivable individuals may harbour clinically significant variants highly specific to other ancestries (‘discordant carriers’). Using local ancestry inference, we identified 177 variants that are exclusive to one ancestral population (‘ancestry-specific variant’), of which 37 were found in 54 discordant carriers. The majority of discordant carriers were R/E-matched (52/54), suggesting cryptic admixture. We found discordant carriers harboured more of the ancestral component linked to the ancestry-specific variant (Fig. 2b , pink bars) than non-carriers for all three ancestral components investigated. For example, the Chinese ancestral component was significantly higher among Indian and Malay carriers of a Chinese-specific variant compared to non-carriers (Fig. 2b left panel, Supplementary Table 5 ), with a median Chinese ancestral component between 28%-32% that is supportive of cryptic admixture. Overall, we were more likely to detect discordant variants (odds ratio (OR): 5.6, 95% confidence interval (CI): 3.11–10.38, p = 6.98 × 10 −10 , two-sided Fisher’s exact test) among individuals with higher levels of genetic admixture (i.e. individuals in the lowest quartile of maxQ values within their ancestry group). Estimates of pathogenic potential among variants of uncertain significance (VUS) Given that deleterious Asian variants are likely to be under-reported or unreported in clinical databases such as ClinVar [34] , we sought to explore potentially pathogenic variants that did not meet our P/LP classification criteria among VUS. We identified missense and cryptic splicing variants with predicted deleterious outcomes using in silico criteria, which we designated as VUS-favour pathogenic (VUS-FP). Among 20,867 VUS with prediction scores, we detected 639 VUS-FP, of which 472 (73.9%) were not reported in ClinVar. Of these, 106 variants occurred in the ACMG SF v3.0 gene list (Supplementary Data 5 ) and we identified an additional 148 individuals with dominantly inherited conditions, translating to an estimated increase in the prevalence of AD conditions in our cohort from 3.41% to 5.05%. We showed that gene-level distribution of variant type tracked the spectrum for known pathogenic variants (Fig. 2c ); for instance, missense VUS-FP were predominantly identified in LDLR and KCNQ1 , genes in which missense variants account for half of the reported disease-associated variants. Using LDLR variants and available low-density lipoprotein (LDL) cholesterol measurements, we evaluated the pathogenicity of VUS-FP. We found that individuals harbouring P/LP and VUS-FP variants were more likely to have clinically high LDL cholesterol levels (defined as ≥4.1 mmol/L by the Ministry of Health Singapore) compared to non-carriers (Fig. 2d ), even after adjusting for age, sex, ancestry and lipid-lowering medication intake (P/LP: OR = 10.83, 95%CI = 4.52–30.05, p = 5.18 × 10 −7 ; VUS-FP: OR = 9.67, 95%CI = 1.41–190.62, p = 0.044). This corroborated our in silico assessment of LDLR VUS-FP, suggesting that VUS-FP account for a proportion of “missing pathogenicity” [35] in under-represented populations. Pharmacogenomic landscape and interaction with genetic disease risk Beyond genetic disease risk, understanding pharmacogenomic diversity, that is variation in the frequency of alleles known to alter an individual’s response to medication, has clinical implications. To examine the pharmacogenomic landscape, we identified known pharmacogenetic alleles of genes in the Clinical Pharmacogenetics Implementation Consortium (CPIC) drug-gene pair list with Pharmacogenomics Knowledgebase (PharmGKB) level 1 evidence. Collectively, 99.7% (9,026/9,051) of SG10K_Health individuals carried at least one actionable pharmacogenetic finding in 23 pharmacogenes with high-confidence gene-drug associations, with a median of five findings per individual. This high frequency is predominantly due to carriers (>98%) of VKORC1 c.−1639G > A (rs9923231) allele affecting sensitivity to the anticoagulant warfarin, which is known to be prevalent among Asians [36] . Of 154 pharmacogenetic variants with actionable phenotype identified (Supplementary Data 6 ), 76.6% (118/154) had a minor allele frequency (MAF) < 1% and 31.8% (49/154) were very rare variants carried by only 1–2 individuals, over half (57.1%, 28/49) of which were found in genes of the cytochrome P450 CYP2 family. Over one-quarter (26.8%, 2429/9051) of our cohort carried a genotype associated with life-threatening drug toxicities including allopurinol- or carbamazepine-induced Stevens-Johnson syndrome/toxic epidermal necrolysis (SJS/TEN, 25.6% HLA-A or HLA-B risk allele carriers), DPD deficiency-linked fluorouracil toxicity (1.4% DPYD intermediate or poor metabolizers) and malignant hyperthermia susceptibility due to potent volatile anaesthetic agents and succinylcholine (0.07% CACNA1S or RYR1 risk allele carriers). Overall, we observed that individuals with actionable pharmacophenotypes associated with commonly prescribed drugs were relatively prevalent, irrespective of ancestry (Table 2 ). Notably, high fractions of individuals were identified with a genotype affecting the activity of cytochrome P450 family of enzymes (Supplementary Data 7 ); for instance 51.0%-77.2% individuals across ancestries harboured alleles associated with actionable phenotypes in CYP2C19 , which is important for metabolism of widely used drugs including the antiplatelet clopidogrel, antiemetics (proton pump inhibitors) and antidepressants such as selective serotonin uptake inhibitors (SSRIs), whereas 31.1–47.2% individuals carried actionable pharmacogenetic variants in CYP2D6 for a broad range of drug interactions including opioids, antidepressants, and tamoxifen therapy for cancer. However, we also found that the prevalence of certain pharmacophenotypes was variable by ancestry; for instance, there were significantly more poor metabolizers among Indians (17.4%) compared to Chinese (3.2%, p = 7.28 × 10 −66 ) and Malays (1.3%, p = 6.50 × 10 −51 ) for UGT1A1 , which metabolizes irinotecan-based drugs frequently used in cancer treatments, due to a higher allele frequency of UGT1A1*28 among Indians. Ancestry-specific variability may also underlie differential genetic profiles for sensitivity to warfarin, which can be attributed to the high frequency VKORC1 rs9923231 among Chinese and Malays as well as the CYP4F2 rs2108622 (c.1297G > A, p.Val433Met) and CYP2C9*3 alleles especially prevalent among Indians (Supplementary Data 6 ). Table 2 Identified alleles in pharmacogenes and the carrier frequency of associated actionable phenotypes among Singaporeans in the SG10K_Health cohort Full size table Next, we explored the intersection of individual genetic disease risk with pharmacogenomic profile by estimating the frequency of individuals harbouring pharmacogenetic variants associated with an actionable phenotype to drugs used for the disorder they are genetically predisposed to. We identified 143 individuals at risk of Centers for Disease Control and Prevention (CDC) Tier 1 genetic conditions (HBOC, Lynch syndrome, FH) [37] , of whom 32 (22.4%) concurrently harboured a pharmacogenetic variant with actionable phenotype to drugs commonly used for treatment of their condition (Fig. 3 , Supplementary Table 6 ). Specifically, 23.0% (14/61) of individuals susceptible to HBOC were also CYP2D6 intermediate or poor metabolizers, who are at higher risk of therapeutic failure for tamoxifen and breast cancer recurrence, whereas eight among 17 individuals with Lynch syndrome predisposition carried either a UGT1A1*6 or UGT1A1*28 allele associated with toxicities related to irinotecan-based chemotherapy. Finally, 15.4% (10/65) of FH-predisposed individuals are concurrently at risk of statin drug-induced myopathies attributed to SLCO1B1 c.521T > C (p.Val174Ala, rs4149056) variant and would benefit from dose adjustment or alternative statins [38] . Fig. 3: Carriers of both germline pathogenic/likely pathogenic (P/LP) variant in a CDC Tier 1 condition and pharmacogenetic variant associated with an actionable phenotype to drugs used for treatment. Only pharmacogenetic variant-drug combinations supported by PharmGKB Level 1A/1B evidence were considered. HBOC hereditary breast and ovarian cancer syndrome, LS Lynch syndrome, FH familial hypercholesterolemia, n number of germline P/LP variant carriers for the indicated CDC Tier 1 genetic conditions among 9051 Singaporeans. Full size image To evaluate for potentially deleterious novel pharmacogenetic variants, we curated for loss-of-function (LOF) variants in 10 of our list of 23 pharmacogenes, whereby LOF is the mechanism associated with actionable phenotype. We identified 47 putative LOF variants, all with a MAF less than 1%. Over half (33/47, 70.2%) of these putative LOF variants are rare, occurring as singletons or doubletons (Supplementary Data 8 ), consistent with the proportions of singleton-doubleton LOF variants reported in whole genome/exome studies from other populations (>58%) [39] , [40] . Notably, half (25/47, 53.2%) of the putative LOF variants were found within the highly polymorphic CYP2C subfamily of cytochrome P450 genes ( CYP2C9, CYPC19, CYP2D6 ), in a total of 95 individuals. The large fraction of rare known risk variants and putative LOF variants identified in pharmacogenes important for metabolizing a broad range of drugs suggests that next-generation sequencing-based assays are warranted for comprehensive pharmacogenetic testing, as genotyping assays may miss or inaccurately detect such rare variants. Here, we characterized clinically significant genetic variation in an ancestrally diverse Southeast Asian population and highlighted diversity in risk profiles for dominant and recessive genetic disorders, capturing the common disorders among Asians missed by prevailing screening panels. Although overall frequency of clinically actionable SFs was comparable to European-centric cohorts, there were differences in concentration of disease burden, exemplified by the higher risk for FH among Chinese in contrast to the higher risk for HBOC among European-descent populations [6] , [41] . Our data also showed that disease risk and carrier burden were varied even among Asian ancestry groups, driven by distinctive prevalence of ancestry-specific recurrent variants. In this study, we characterized genetic risk in Malays, a severely under-represented Austronesian-speaking Southeast Asian population, and highlighted distinction in their disease risk profiles compared to East and South Asians. Emblematic of current Eurocentric genomic medicine guidelines, we found 27% of severe recessive disorder genes with carrier frequencies exceeding 1-in-200 Asians are unrepresented in ACMG carrier screening recommendations or commercial carrier screening panels. Left unaddressed, Asian couples will be at greater risk for conditions missed by existing screening panels and based on our lower-bound estimate of 0.51% Singaporean ARCs for severe recessive disorders, conservative projection to a combined reproductive-age population of 94 million encompassing South India, South China and Austronesian-speaking Southeast Asia would translate to almost half a million at-risk Asian couples standing to benefit from carrier screening. This is slightly lower compared to the ARC rate of 0.8%-1.0% observed in a population of Estonian and Dutch couples of European ancestry [42] and is likely due to the under-reporting of Asian variants in clinical databases and literature [43] , [44] . Our findings underscore the importance of diverse representation in genetic risk profiling across disease domains and in development of clinical recommendations, particularly within multi-ethnic settings, to address disparities in health care delivery and outcomes. Cross-ancestry differences extend beyond disease prevalence to the spectrum of genetic variants for the same gene, potentially accounting for inter-population variability in disease manifestation. For instance, the GJB2 c.35delG (p.Gly12Valfs*2) variant associated with profound hearing loss is prevalent among populations of European-descent [22] but rare among Asians of Chinese and Malay ancestry, most of whom harbour the Val37Ile variant associated with mild-to-moderate hearing impairment. Notably, whereas cystic fibrosis is prevalent in European-descent populations and frequently associated with CFTR c.1521_1523delCTT (p.Phe508del) variant, this is rare in Asia where CFTR -related CBAVD and pancreatitis are more frequently observed together with CFTR c.1210-11T > G and Gln1352His variants [45] , [46] . Under-recognition of such genotype-phenotype associations can have consequences, as symptoms for less-characterized disorders afflicting non-European groups may go undetected and result in misdiagnosis or missed opportunities for early intervention. The prevalence of cryptic admixture in our multi-ethnic cohort highlights the pitfalls of over-reliance on self-reported R/E for genetic risk profiling [5] , [12] . Notably, we observed a self-identified Chinese adult female carrying a Malay founder variant for BRCA1 (Asn909Lysfs*6) [20] , [47] as well as numerous Chinese and Indian individuals harbouring variants identified recurrently among Malays (e.g. ABCA4 Arg24His, ARHGEF18 c.826-1G > A); all of whose genetic ancestry includes an appreciable (10%-20%) Malay ancestral component. This is consistent with Singapore’s history of immigration, epitomized by admixture among the Peranakan community established through inter-marriage between Chinese and Indian immigrants with native Malays since the 15th century [48] . Our findings highlight that genetic susceptibility to health disorders cuts across ethnic boundaries, especially as populations become increasingly admixed worldwide, driven by intercontinental unions and human migration accelerated by socio-geopolitical factors. With Asians accounting for the rapid rise in minority/immigrant groups in the United States and Europe [49] , [50] , integration of Asian population-derived data will be increasingly relevant for more precise clinical risk assessment and narrowing gaps in health care delivery. At present, the ‘informational disparity’ stemming from Eurocentric studies [11] limits clinical interpretation of variants detected in under-represented ancestry groups and as indicated by our data, there are Asian-specific pathogenic variants that are currently classified as VUS, which can be reclassified with increased detection through widespread testing. Our study comprehensively profiled high confidence gene-drug interactions across three Asian ancestries, using whole-genome sequencing to uniformly analyse the pharmacogenomics of a large cohort of these ancestries. We demonstrated contrasting drug response profiles along ancestry lines driven by variability in allele frequencies, consistent with a smaller Singaporean study [51] , contributing to distinctive pharmacologic susceptibility across ancestry groups. Importantly, we showed that approximately one-fifth of individuals with predisposition to a genetic disorder are at risk of therapeutic failure or life-threatening toxicity for drugs commonly prescribed to treat the disease. This highlights that a substantial fraction of genetically susceptible individuals could benefit from pre-emptive pharmacogenomics to optimize their therapeutic treatments and avoid severe toxicities, indicating opportunities to forge a more comprehensive clinical care by combining pharmacogenomics and genetic disease testing. This work demonstrates that Asians are a diverse population with complex genomic architecture and extensive genetic variability. Although a conservative estimate of Asian population genetic risk given the focus on known disease genes and coding variants, our data provides opportunities to address disparities in existing knowledge by demonstrating the contrast in risk profiles of monogenic disorders between European and Asian ancestry groups and the need for expanded carrier testing among Asians. Beyond diversity, we also showed that monogenic disorder pathogenic variants are mostly rare, with >85% carried in only 1–2 individuals, supporting the need for comprehensive sequence-based testing as opposed to array-based single nucleotide polymorphism (SNP) genotyping [52] . Critically, we highlighted the prevalence of cryptic admixture and limitation of self-reported R/E in estimating genetic risk burden in an ethnically diverse population and demonstrated the potential benefit of coupling pharmacogenomics with clinical genetic testing. As genomic profiling gains traction in mainstream precision medicine, the diversified representation of all population groups in genomic research will be imperative to level the gaps in health disparity for a truly equitable delivery of precision medicine. Study population The source dataset used for this study was derived from the SG10K_Health project. Individuals from six participating studies (Supplementary Table 1 ) were recruited with signed informed consent from the participating individual or parent/guardian in the case of minors. Germline DNA for whole genome sequencing were extracted from whole blood or cord blood (for birth cohort) specimens of enrolled individuals according to respective study protocols. All studies were approved by relevant institutional ethics review board detailed in Supplementary Table 1 . The final analysed cohort comprised 9051 individuals inferred to be unrelated to the second degree through kinship analysis, with global genetic ancestry (henceforth, ‘genetic ancestry’) inferred through admixture analysis (subsection: Kinship and admixture inference). For ancestry analysis, self-reported race/ethnicity (R/E) was captured from the respective national identification document of participating individuals. Sequencing and bioinformatics analysis We performed whole genome sequencing for germline DNA on Illumina Hiseq X platform to a target depth of 30X or 15X. Resulting paired-end sequencing reads were jointly-processed in a standardized bioinformatics pipeline that involved alignment to the human reference genome (hg38) using Burrows-Wheeler Aligner (BWA-MEM, v0.7.17) [53] followed by GenomeAnalysisToolKit (GATK, v4.0.6.0) best practices workflow to produce a jointly-genotyped variant call file (VCF) comprising 9,770 samples [54] , [55] . To accelerate variant annotation, we trimmed the full VCF to retain only positions overlapping our genes list (subsection: Gene selection) and samples that were unrelated up to the seconds degree ( n = 9,051). Heterozygous sites were re-genotyped to “no call” status if the following criteria were unmet: (1) allele balance between 20% and 80%, (2) minimum read depth of 5, (3) minimum genotype quality of 20. We performed variant annotation using Ensembl Variant Effect Predictor (VEP, release 100.0) [56] to include information such as overlapping genes, consequence type, Human Genome Variation Society (HGVS) nomenclature for DNA and protein alterations, population allele frequencies and in silico pathogenicity prediction scores from REVEL (rare exome variant ensemble learner) [57] , PrimateAI [58] and SpliceAI [59] . As VEP provides one predicted consequence for each transcript, we selected the consequence on the MANE (Matched Annotation from NCBI and EMBL-EBI) transcript. Where a gene does not have a MANE transcript, the transcript with the most deleterious variant consequence and/or the longest gene transcript affected was selected. Samples sequenced to target depth of 30X versus 15X were evaluated for potential batch effects and the carrier frequencies of identified variants were shown to be strongly correlated (Pearson’s r > 0.86, Supplementary Fig. 5 ). Gene selection We consolidated a list of 4143 genes (Supplementary Data 9 ) associated with autosomal dominant (AD), autosomal recessive (AR), and X-linked monogenic disorders from three sources: (1) 3252 genes with diagnostic-grade (green) status from PanelApp [60] (accessed 5 May 2020), (2) 5,506 genes from Online Mendelian Inheritance in Man (OMIM) ( www.omim.org , accessed 21 May 2020), (3) 4121 genes from in-house gene panels for cardiomyopathies, cancer predisposition, paediatrics and ophthalmology. We excluded genes linked to repeat expansion disorders. Identification of loss-of-function intolerant (LOFi) genes We defined a total of 1,856 genes as LOFi if any one of the following criteria was fulfilled: (1) genes considered to be haploinsufficient by the Clinical Genome Resource [61] (ClinGen, n = 727, accessed May 01 2020), (2) genes with ≥3 variants classified as pathogenic or likely pathogenic in ClinVar [62] with a review status of at least 2 gold stars (i.e. is a practice guideline, or has been reviewed by expert panel, or has multiple submitters with criteria provided and no conflicts; subsequently referred to as ‘ClinVar TwoPlus’ variants) and were one of the following variant types: frameshift insertion/deletion, nonsense, essential splice site variant (±2 residues from splice site) ( n = 587, accessed September 09, 2020), (3) genes with ExAC pLI [63] (probability of being LOFi, obtained from dbNSFP 4.0) score > 0.9 ( n = 983). Variant classification and interpretation We retained variants that overlapped genes in our consolidated gene list for curation if reported in ClinVar or had a SG10K_Health allele frequency <0.05, and were categorised into one of the following groups (Supplementary Fig. 1 ): (1) Pathogenic/Likely Pathogenic (P/LP), (2) Variants of uncertain significance-favour pathogenic (VUS-FP), (3) Variants of uncertain significance (VUS), (4) Unclassified. Pathogenic/Likely Pathogenic (P/LP) We further subset variants in this group into three categories: (1) Tier1A_TwoPlus: ClinVar TwoPlus variants were considered high confidence known pathogenic variants and automatically classified as P/LP. Novel single nucleotide variants that result in known amino acid codon change that has a ClinVar TwoPlus status were also categorized as P/LP. (2)Tier1A_Conflicting: Variants in ClinVar with conflicting interpretations but ≥4P/LP submissions were considered P/LP whereas those with 1-3P/LP submissions were manually curated according to American College of Medical Genetics and Genomics and the Association for Molecular Pathology (ACMG/AMP) guidelines [64] , taking into consideration allele frequency, in silico scores and reports in literature (Human Gene Mutation Database (HGMD) [65] and PubMed). Known variants that occurred in cis such as GAA c.752C > T;c.761 C > T were counted as one event. (3) Tier1B: LOF variants (frameshift insertions/deletions, nonsense, essential splice site variants) that were either absent in ClinVar or that were in ClinVar but did not meet our preceding criteria, were manually curated according to the ACMG/AMP PVS1 criterion using the high-throughput, automated application AutoPVS1 (v1.1) [66] . Variants fulfilling the following criteria were considered P/LP: (a) LOF consequence in MANE transcript; for genes without MANE transcript, ClinVar and the National Center for Biotechnology Information (NCBI) were referenced to determine the LOF variant affected a clinically relevant transcript, and (b) AutoPVS1 indicated PVS1 strength of “Very Strong”, or (c) there are ≥2 ClinVar TwoPlus P/LP variants located downstream of the variant. Truncating variants in TTN were separately assessed using CardioClassifier [67] (v.0.2.0) for P/LP classification. Variants of uncertain significance (VUS) and VUS-favour pathogenic (VUS-FP) Variants that did not meet our P/LP criteria were considered VUS. We also considered the following variants as VUS: (1) Variants in ClinVar with conflicting interpretations but ≥4 VUS submissions, (2) LOF variants in close proximity, which upon manual inspection using Integrative Genomics Viewer (IGV, v2.8.2) [68] showed a non-frameshift insertion/deletion consequence. We defined VUS with potential LOF consequence as VUS-FP if the following criteria were met: (a) missense variants with REVEL score >0.7 and are located in a ‘hotspot’ (defined as a rolling window of 25 bp with >2 ClinVar TwoPlus P/LP variants and with the number of benign/likely benign variants less than ClinVar TwoPlus P/LP variants), or (b) cryptic splice variants with SpliceAI maximum score >0.8 and occurred in genes with ≥5 ClinVar TwoPlus P/LP LOF (nonsense/frameshift/canonical splice) variants. All remaining variants that did not meet any of the P/LP, VUS or VUS-FP criteria were categorised as “Unclassified”. Gross deletions We derived gross deletions included for our analysis from a structural variant (SV) callset generated by the SG10K_SV workgroup. For each sample, CRAM file was processed using Manta (v1.6) [69] to identify candidate SVs. Subsequently, the SVs across all samples were merged using svimmer (v0.1), and then re-genotyped using graphtyper2 (v2.5.1) [70] . To identify high-confidence CNVs, duphold (v0.2.3) [71] was performed to add read-depth information to the SV calls. We considered only deletions that overlapped at least an exon of the MANE transcript in our LOFi gene list and that met the following criteria: (1) length of 500 bp–10 Mbp, (2) deletions with duphold DHFC, DHFFC, DHBFC values <0.7 and DHSP > 1. We visually confirmed candidate CNVs using samplot (v1.0.20) [72] . We separately identified deletions in SMN1 using SMNCopyNumberCaller (v1.1.1) [73] only on samples with 30X sequencing coverage. Virtual mating simulation To estimate frequency of at-risk couples (ARCs) for recessive disorders, we considered all possible matings within each ancestry group, regardless of sex [42] (Chinese, CH = 15,133,251; Indian, IND = 1,882,770; Malay, MY = 1,292,028). We considered a simulated couple to be at-risk if both carried P/LP variants in one or more AR genes associated with severe recessive disorder [32] . We created an exclusion list comprising variants considered to cause clinically significant disease only in trans with a more severe P/LP variant, hence if a theoretical couple were simulated to have an offspring that is homozygous for a variant in the exclusion list or compound heterozygous for two variants within the exclusion list, the couple was not considered to be an ARC. Kinship and admixture inference To perform kinship analysis, we extracted a set of known polymorphic sites from the full VCF using Somalier (v0.2.13) [74] and processed using PLINK (v1.90b3.46) [75] to produce a PLINK BED reference panel, consisting single nucleotide polymorphisms (SNPs) pruned with r 2 > 0.5 (using PLINK recommended settings of window sizes of 50 SNPs with steps of 5 SNPs across the genome). We used Kinship-based Inference for Genome-wide association studies (KING, ver 2.2.3) [76] to calculate pairwise kinship coefficients and considered pairs of samples with kinship coefficient ≥0.0884 as related, and randomly select one from each pair for exclusion. For global ancestry inference, we performed admixture analysis to estimate the proportions of three hypothetical ancestral components in each sample on ADMIXTURE (ver 1.3.0) [15] with K = 3 using the same PLINK BED reference panel. The hypothetical components of K = 3 has been demonstrated to sufficiently delineate the three major ancestry groups (Chinese, Indian, Malay) in a Singaporean cohort [14] . The highest of the three estimated ancestral components for each individual was inferred as genetic ancestry. For the purpose of our analyses, “genetic ancestry” assigned to each individual is a statistical construct calculated from inherited genetic variants and is not equivalent to, nor intended to replace, self-reported race or ethnicity, which are social constructs identified by the individuals. To estimate local ancestry, we used phased genotypes generated using EAGLE (v2.4.1) and retained only SNPs with minor allele frequency ≥ 1% and call rate of ≥ 0.5. We selected 100 individuals from each ancestry group with the highest respective ancestral component, and the combined 300 individuals representing Chinese, Indian and Malay ancestry groups were used as the reference panel for inference of local ancestry using RFMix (v2.03-r0) [77] on default settings. In the analysis of discordant variant carriers in Fig. 2b , we defined ancestry-specific variants by the following criteria: (1) P/LP variants with allele count ≥5, and (2) the variant exclusively occurs in an allele with the same inferred local ancestry. For instance, a Chinese-specific variant is one that occurs exclusively in alleles with inferred local ancestry of Chinese origin. Pharmacogenomic variants For profiling the pharmacogenomic landscape, we consolidated a list of 23 pharmacogenes from the CPIC (Clinical Pharmacogenetics Implementation Consortium) drug-gene pair list (Supplementary Data 10 , accessed Aug 30 2021) with Pharmacogenomics Knowledgebase (PharmGKB) clinical annotation level of evidence 1A/1B, which are defined as: (Level 1A) gene-drug combinations with variant-specific prescribing guidance in existing clinical guideline annotation or an FDA-approved drug label annotation, and minimally one publication supporting the clinical annotation, or (Level 1B) gene-drug combinations with no variant-specific prescribing guidance but has a high level of evidence supporting the association with at least two independent publications [78] . Referencing the CPIC and Pharmacogene Variation Consortium (PharmVar) repositories (accessed April 2021), we identified known pharmacogenetic alleles of these 23 genes using the following methods: (a) Cyrius (v1.0) [79] ( CYP2D6 ) and Aldy (v3.1) [80] for genes with star allele nomenclature, (b) HLA-HD (v1.3.0) [81] for HLA-A and HLA-B alleles, (c) VCF-derived for genes with pharmacogenetic alleles defined by dbSNP rsIDs. Allele frequencies for each allele with a functional status associated with known pharmacogenetic phenotype is tabulated in Supplementary Data 6 , whereas the carrier frequency of actionable pharmacogenetic phenotypes associated with the 23 pharmacogenes is tabulated in Table 2 , and further consolidated by actionable phenotype with therapeutic recommendation guidelines in Supplementary Data 7 . Carrier frequency for diplotypes associated with actionable phenotypes for pharmacogenes with star nomenclature is consolidated in Supplementary Data 11 . For identification of potentially deleterious novel variants (i.e. not found in CPIC or PharmVar), we filtered for putative LOF variants (frameshift insertions/deletions, nonsense, essential splice site) that: (a) are located in MANE transcript, and (b) AutoPVS1 indicated PVS1 strength of “Very Strong”, and (c) occurred in 10 of the 23 pharmacogenes in our list, for which LOF is a mechanism associated with the actionable phenotype ( CYP2B6, CYP2C9, CYP2C19, CYP2D6, DPYD, G6PD, NUDT15, SLCO1B1, TPMT, UGT1A1 ). Upon manual review, one variant ( SLCO1B1 c.1738C > T (p.Arg580*), rs71581941) was removed due to poor read coverage. Statistical analysis We performed all statistical analyses using R version 4.1.0 [82] . Cohort data, gene- and variant-level carrier frequencies were tabulated with descriptive statistics. We performed two-sided Fisher’s exact test for comparison of proportions for categorical variables, whereas two-sided Wilcoxon rank-sum test was used for comparing continuous variables. p values were adjusted with Benjamini-Hochberg correction for multiple testing. Binomial logistic regression was used for comparison of LDL cholesterol levels against LDLR variant status, correcting for age, sex, ancestry and lipid-lowering medication intake. Reporting summary Further information on research design is available in the Nature Research Reporting Summary linked to this article.